Mediator MED23 cooperates with RUNX2 to drive osteoblast differentiation and bone development How lineage specifiers are regulated during development is an outstanding question, and the molecular regulation of osteogenic factor RUNX2 remains to be fully understood. Here we report that the Mediator subunit MED23 cooperates with RUNX2 to regulate osteoblast differentiation and bone development. Med23 deletion in mesenchymal stem cells or osteoblast precursors results in multiple bone defects similar to those observed in Runx2 +/− mice. In vitro , Med23 -deficient progenitor cells are refractory to osteoblast differentiation, and Med23 deficiency reduces Runx2 -target gene activity without changing Runx2 expression. Mechanistically, MED23 binds to RUNX2 and modulates its transcriptional activity. Moreover, Med23 deficiency in osteoprogenitor cells exacerbates the skeletal abnormalities observed in Runx2 +/− mice. Collectively, our results establish a genetic and physical interaction between RUNX2 and MED23, suggesting that MED23 constitutes a molecular node in the regulatory network of anabolic bone formation and related diseases. Mesenchymal stem cells (MSCs) are multipotent progenitors that can self-renew and differentiate into several distinct cell lineages, including osteoblasts, chondrocytes and adipocytes [1] , [2] . Their differential potentials and intrinsic properties make MSCs of great interest for applications in a variety of cell-based therapies [3] , [4] , [5] , [6] . In the past few decades, several master regulators that specify the various cell fates associated with MSCs have been identified: for example, Runx2 triggers MSCs to differentiate into osteoblasts [7] , [8] . The function of Runx2 in osteoblast differentiation was initially demonstrated by observations that Runx2 −/− mice lack both mature osteoblasts and a mineralized skeleton [8] , [9] , [10] . Although Runx2 +/− mice do undergo skeletal mineralization, the process is impaired, with delayed closure of the fontanelles and clavicular hypoplasia [10] , resembling the cleidocranial dysplasia (CCD) phenotype that arises from Runx2 haploinsufficiency in humans [9] . The skeletal pathologies in humans and mice highlight the importance of the precise regulation of Runx2 activity during osteogenesis. Apart from these key transcription factors, several cofactors have been found to be involved in the fine tuning of cell-fate determination [11] , [12] , [13] . One such cofactor is the transcriptional complex Mediator, which is a multiprotein complex that has been evolutionarily conserved from yeast to metazoans. The Mediator complex is recruited by transcription factors in response to developmental or environmental signals. Through direct protein interactions, Mediator links transcription factors to the RNA polymerase II (Pol II) machinery and modulates the transcriptional output [14] . Our previous research demonstrated that the Mediator MED23 subunit acts as a molecular modulator to control the balance between adipogenesis and myogenesis [15] , [16] . However, it remained unknown whether MED23 is also involved in the development of osteoblasts, which, like adipocytes and myocytes, are also derived from mesenchymal progenitors. In this study, we provide evidence of a role for MED23 in osteogenesis. Mice deficient in Med23 in MSCs or preosteoblasts display defective bone formation and impaired osteoblast differentiation, resembling the skeletal phenotype of Runx2 +/− mice. Further molecular studies demonstrate that MED23 cooperatively interacts with RUNX2 in the regulation of osteogenesis. Our results reveal that MED23 is an important regulator of osteogenesis and is essential for the transcriptional activity of RUNX2. Med23 deficiency in MSCs impaired bone ossification To investigate the role of Med23 in the commitment of MSCs to an osteoblast fate, we generated a Med23 conditional knockout mouse model by crossing Med23 fl/fl mice [17] with Prx1-Cre mice ( Fig. 1a ). The latter is a transgenic line wherein Cre activity is largely confined to ventral and craniofacial mesenchyme [18] , [19] . Western blot assays verified that MED23 was largely abrogated in bone marrow-derived MSCs ( Fig. 1b ). MSC-specific Med23 deletion had no effect on survival or fertility. However, Med23 fl/fl ; Prx1-Cre mice ( Med23 MSC −/− ) were shorter and underweight relative to their control littermates. Furthermore, as the Med23 MSC −/− mice aged, they developed a marked dwarfism phenotype with short legs that was independent of sex ( Fig. 1c,d ). The heterozygous mice ( Med23 MSC +/− ) appear normal (Supplementary Fig. 1d). Consistent with this observation, the level of MED23 was barely reduced in bone tissue samples from Med23 MSC +/− mice (Supplementary Fig. 1c). 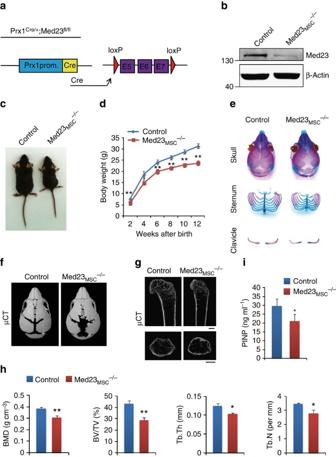Figure 1: Inactivation ofMed23in mesenchymal stem cells causes impaired bone ossification. (a) Illustration ofMed23deletion in Prx1-expressing mesenchymal stem cells. (b) Expression ofMed23protein in bone marrow-derived mesenchymal stem cells from 6- to 8-week-old control (Med23fl/fl) andMed23MSC−/− mice. (c) Representative view of 1-month-old control andMed23MSC−/−mice. (d) Body weight of male control mice andMed23MSC−/−littermates measured at different age points (n=3 for each group,t-test). Data represent means±s.d. *P<0.05, **P<0.01. (e) Skeletal preparations from control andMed23MSC−/−newborns were double stained with Alizarin red and Alcian blue. (f) Microcomputed tomography (μCT) image of skulls from control andMed23MSC−/−mice at postnatal day 6 (P6). (g) μCT images of distal femurs from 1-month-old control andMed23MSC−/−mice (top panel, longitudinal view; bottom panel, axial view of the metaphyseal region). Scale bar, 1 mm. (h) Quantitative μCT analysis of distal femurs from 1-month-old control (n=5) andMed23MSC−/−mice (n=4), including bone mass density (BMD), bone volume per tissue volume (BV/TV), trabecular thickness (Tb.Th) and trabecular number (Tb.N). Data represent means±s.e.m.t-test,*P<0.05, **P<0.01. (i) ELISA analysis of serum PINP (ng ml−1) from 1-month-old control andMed23MSC−/−mice (n=4). Data represent means±s.d.t-test, *P<0.05, **P<0.01. Figure 1: Inactivation of Med23 in mesenchymal stem cells causes impaired bone ossification. ( a ) Illustration of Med23 deletion in Prx1-expressing mesenchymal stem cells. ( b ) Expression of Med23 protein in bone marrow-derived mesenchymal stem cells from 6- to 8-week-old control ( Med23 fl/fl ) and Med23 MSC −/− mice. ( c ) Representative view of 1-month-old control and Med23 MSC −/− mice. ( d ) Body weight of male control mice and Med23 MSC −/− littermates measured at different age points ( n =3 for each group, t -test). Data represent means±s.d. * P <0.05, ** P <0.01. ( e ) Skeletal preparations from control and Med23 MSC −/− newborns were double stained with Alizarin red and Alcian blue. ( f ) Microcomputed tomography (μCT) image of skulls from control and Med23 MSC −/− mice at postnatal day 6 (P6). ( g ) μCT images of distal femurs from 1-month-old control and Med23 MSC −/− mice (top panel, longitudinal view; bottom panel, axial view of the metaphyseal region). Scale bar, 1 mm. ( h ) Quantitative μCT analysis of distal femurs from 1-month-old control ( n =5) and Med23 MSC −/− mice ( n =4), including bone mass density (BMD), bone volume per tissue volume (BV/TV), trabecular thickness (Tb.Th) and trabecular number (Tb.N). Data represent means±s.e.m. t -test,* P <0.05, ** P <0.01. ( i ) ELISA analysis of serum PINP (ng ml −1 ) from 1-month-old control and Med23 MSC −/− mice ( n =4). Data represent means±s.d. t -test, * P <0.05, ** P <0.01. Full size image Notably, the membranous ossification of the skull was impaired in Med23 MSC −/− newborns compared with control littermates. The anterior and posterior fontanelles were enlarged and the cranial sutures were wider in Med23 MSC −/− mice. Defective osteogenesis was not limited to cranial tissues, as the clavicles became thinner and shorter, and the sternum xiphoid was also hypoplastic ( Fig. 1e ). And these defects occurred as early as E15.5 when the bone mass is formed (Supplementary Fig. 1a). By contrast, a skeletal analysis of Med23 MSC +/− mice confirmed that they were phenotypically normal relative to control littermates (Supplementary Fig. 1b). To further determine the function of MED23 in the skeletal system, we utilized micro-quantitative computed tomography micro computed tomography (μ-CT) to compare skeletal elements isolated from Med23 MSC −/− mice with corresponding elements from control littermates. As shown in Fig. 1f , 6-day-old Med23 MSC −/− mice displayed hypomineralization of the calvaria compared with control mice. In addition, we found that 1-month-old Med23 MSC −/− mice were osteopenic, with reduced bone mineral density (BMD) and bone volume per tissue volume) (BV/TV) in the femoral trabecular bone relative to age-matched control littermates. Further analysis showed that the reduced trabecular number (Tb.N) of Med23 MSC −/− mice was accompanied by decreased trabecular thickness (Tb.Th) and a reduction in the Tb.N compared with those of control mice ( Fig. 1g,h ). Consistent with the decreased BMD in Med23 MSC −/− mice, an ELISA assay of PINP (N-terminal propeptide of type I procollagen), a marker of bone formation, revealed a reduced bone formation rate in Med23 MSC −/− mice ( Fig. 1i ). In adults, bone is continuously remodelled by bone-resorbing osteoclasts and bone-forming osteoblasts [20] . We performed a histological analysis and in vitro osteoclastogenesis experiment to exclude the possibility that the decreased bone density in the long bones of Med23 MSC −/− mice could be attributed to increased osteoclast differentiation and/or activity. We found that osteoclast activity was comparable between Med23 MSC −/− mice and their control littermates (Supplementary Fig. 2a,b). Moreover, the expression of osteoclastic genes did not change either (Supplementary Fig. 2c). Taken together, these results suggest an important role for Med 23 in bone formation. Ablation of Med23 in preosteoblasts reduced bone formation To further determine whether the abnormal osteogenesis in Med23 MSC −/− mice results from a primary defect in osteoblast development, we generated an osteoblast-specific Med23 -deleted mouse model ( Med23 ob −/− mice) by crossing Med23 fl/fl mice with osterix ( Osx ) -Cre mice, a line in which Cre expression is primarily restricted to osteoblast precursors [21] ( Fig. 2a ). Western blot assays showed that MED23 decreased in the bone of both Med23 ob +/− and Med23 ob −/− mice (Supplementary Fig. 3b). Consistent with decline in protein of MED23, histological analysis by alcian blue and alizarin red (ARS) staining showed defects in the skeleton occurring in both Med23 ob +/− and Med23 ob −/− newborns, and more severe in the latter, including abnormality in calvarial and clavicle ossification (Supplementary Fig. 3a). However, Osx -Cre transgenic mice have been found to manifest defects in bone phenotype, such as to delay bone mineralization and develop scapula calluses [22] , [23] . To exclude such effect of Osx-Cre, we made a comparison between Med23 ob −/− mice and Med23 ob +/− control littermates that were both in the context of Osx -Cre. Again, Med23 ob −/− mice developed runty and underweight compared with age-matched control littermates ( Fig. 2b,c ). Mice with Med23 deficiency in osteoblast reproduced the phenotype of Med23 MSC −/− mice, including impaired membranous ossification of calvarial bones and dysplasia of the clavicles, although the sternum appeared normal. In the Med23 ob −/− mice, the bone was obviously porous; this feature was more evident in the bones of the skull ( Fig. 2d,e ). μCT analysis further confirmed the osteopenic phenotype of Med23 ob −/− mice ( Fig. 2f,g ). Likewise, relatively lower levels of serum PINP indicated a decreased bone formation rate in Med23 ob −/− mice ( Fig. 2h ). Again, in vivo and in vitro osteoclastogenesis showed comparable levels of osteoclasts between Med23 ob −/− mice and control littermates (Supplementary Fig. 4a–c). Hence, the Med23 ob −/− mice recapitulate the defects observed in Med23 MSC −/− mice with striking fidelity, supporting the conclusion that Med23 is necessary to the differentiation and function of committed osteoblast precursors. 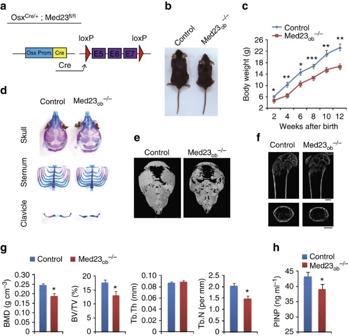Figure 2: Inactivation ofMed23in osteoblast progenitors results in defects in bone formation. (a) Illustration ofMed23deletion inOsx-expressing osteoblast progenitors. (b) Representative view of 1-month-old control (Med23ob+/−) andMed23ob−/−mice. (c) Body weight of male control mice andMed23ob−/−littermates measured at different age points (n=3). Data represent means±s.d.t-test, *P<0.05, **P<0.01, ***P<0.001. (d) Skeletal preparations from control andMed23ob−/−newborns were double stained with Alizarin red and Alcian blue. (e) μCT image of skulls from control andMed23ob−/−mice at postnatal day 6 (P6). (f) μCT images of distal femurs from 1-month-old control andMed23ob−/−mice. Scale bar, 1 mm. (g) Quantitative μCT analysis of trabecular bone in the distal femurs from 1-month-old control andMed23ob−/−mice (n=3). Data represent means±s.e.m.t-test, *P<0.05. (h) ELISA analysis of serum PINP (ng ml−1) from 1-month-old control andMed23ob−/−mice (n=4). Data represent means±s.d.t-test, *P<0.05. Figure 2: Inactivation of Med23 in osteoblast progenitors results in defects in bone formation. ( a ) Illustration of Med23 deletion in Osx -expressing osteoblast progenitors. ( b ) Representative view of 1-month-old control ( Med23 ob +/− ) and Med23 ob −/− mice. ( c ) Body weight of male control mice and Med23 ob −/− littermates measured at different age points ( n =3). Data represent means±s.d. t -test, * P <0.05, ** P <0.01, *** P <0.001. ( d ) Skeletal preparations from control and Med23 ob −/− newborns were double stained with Alizarin red and Alcian blue. ( e ) μCT image of skulls from control and Med23 ob −/− mice at postnatal day 6 (P6). ( f ) μCT images of distal femurs from 1-month-old control and Med23 ob −/− mice. Scale bar, 1 mm. ( g ) Quantitative μCT analysis of trabecular bone in the distal femurs from 1-month-old control and Med23 ob −/− mice ( n =3). Data represent means±s.e.m. t -test, * P <0.05. ( h ) ELISA analysis of serum PINP (ng ml −1 ) from 1-month-old control and Med23 ob −/− mice ( n =4). Data represent means±s.d. t -test, * P <0.05. Full size image Med23 is required for the osteoblast differentiation of MSCs Next, we asked whether Med23 deficiency affects the osteogenic potential of MSCs in a cell-autonomous manner. Primary MSCs were isolated from the bone marrow of control and Med23 MSC −/− littermates, and the deficiency of Med23 in the MSCs from Med23 MSC −/− mice was confirmed by western blot assay ( Fig. 3a ). Med23 deficiency in MSCs does not appear to alter the cell viability or growth rate, indicated by comparable numbers of colony-forming unit fibroblasts (c.f.u.-F) ( Fig. 3b ). However, Med23 −/− MSCs displayed markedly decreased alkaline phosphatase (ALP) activity and mineralization ( Fig. 3c,d ). In addition, the mRNA levels of osteogenic genes, such as osteocalcin ( Ocn ), were significantly downregulated in Med23 MSC −/− cells ( Fig. 3e ), while Runx2, a key regulator in bone development, did not change during osteogenesis ( Fig. 3a,e ). Similarly, impaired osteogenesis was observed in Med23-deficient osteoblasts too (Supplementary Fig. 6). These results indicated that Med23 functioned necessarily in osteogenesis in vitro . 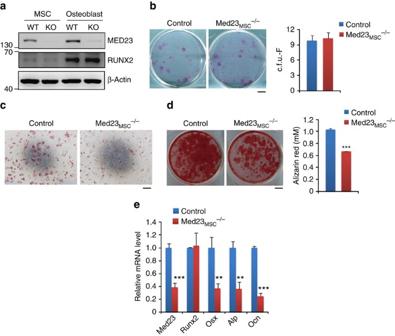Figure 3: Med23 deficiency inhibits osteoblast differentiation. (a) Expression of Med23 and Runx2 in bone marrow-derived mesenchymal stem cells and calvarial osteoblasts from 6 to 8-week-old control andMed23MSC−/−mice. Isolated cells were expanded and analysed by western blotting. (b) c.f.u.-F assay for bone marrow cells from control andMed23MSC−/−littermates. Representative images of c.f.u.-Fs stained with crystal violet (left, scale bar, 0.5 cm) and quantification of c.f.u.-Fs (right,n=3 for each group.). Data represent means±s.d.t-test. (c) ALP staining of bone marrow mesenchymal stem cells after cultured for 7 days in osteogenic medium. Scale bar, 500 μm. (d) c.f.u.-ob assay for bone marrow of control andMed23MSC−/−littermates. Bone marrow cells were cultured in osteogenic medium for 21 days, followed by staining with Alizarin red (left, scale bar, 0.5 cm) and quantification (right,n=3 for each group). Data represent means±s.d.t-test.***P<0.001 (e) The relative mRNA levels ofMed23,Runx2,Osx,AlpandOcnwere quantified by RT–PCR. Data represent means±s.d. All data represent means±s.d.t-test, **P<0.01, ***P<0.001. Figure 3: Med23 deficiency inhibits osteoblast differentiation. ( a ) Expression of Med23 and Runx2 in bone marrow-derived mesenchymal stem cells and calvarial osteoblasts from 6 to 8-week-old control and Med23 MSC −/− mice. Isolated cells were expanded and analysed by western blotting. ( b ) c.f.u.-F assay for bone marrow cells from control and Med23 MSC −/− littermates. Representative images of c.f.u.-Fs stained with crystal violet (left, scale bar, 0.5 cm) and quantification of c.f.u.-Fs (right, n =3 for each group.). Data represent means±s.d. t -test. ( c ) ALP staining of bone marrow mesenchymal stem cells after cultured for 7 days in osteogenic medium. Scale bar, 500 μm. ( d ) c.f.u.-ob assay for bone marrow of control and Med23 MSC −/− littermates. Bone marrow cells were cultured in osteogenic medium for 21 days, followed by staining with Alizarin red (left, scale bar, 0.5 cm) and quantification (right, n =3 for each group). Data represent means±s.d. t -test. *** P <0.001 ( e ) The relative mRNA levels of Med23 , Runx2 , Osx , Alp and Ocn were quantified by RT–PCR. Data represent means±s.d. All data represent means±s.d. t -test, ** P <0.01, *** P <0.001. Full size image To exclude developmental differences between control and Med23 −/− primary MSCs, we infected wild-type primary bone marrow MSCs with retroviruses expressing either shRNAs targeting Med23 or control shRNA. Consistent with the differentiation difference between WT and Med23 KO primary MSCs, shRNA-mediated acute knockdown of Med23 in MSCs also resulted in decreased osteogenesis, as indicated by ALP and ARS staining (Supplementary Fig. 5a). Real-time PCR analysis showed that Med23 knockdown reduced the expression of osteogenic marker genes such as Osx , Alp , collagen type I ( Col1a1 ) and Ocn . However, noticeably, the expression of Runx2, the master regulator for osteoblast differentiation, was unaffected by Med23 deficiency (Supplementary Fig. 5b). Collectively, these results showed that Med23 is required for osteoblast differentiation. The key osteogenic genes downregulated in Med23 -deficient cells are known targets of Runx2, suggesting that MED23 might regulate osteoblast differentiation via Runx2. Med23 regulates the gene network of bone development Despite our observation that the expression of Runx2 , a master transcription factor for osteoblast differentiation, was not affected by Med23 deletion during osteogenesis, Med23 MSC −/− mice appeared to phenocopy the skeletal defects of Runx2 +/− mice, including delayed closure of the fontanelles, clavicular hypoplasia and decreased bone density [10] , suggesting that Med23 and Runx2 share a functional mechanism. To compare the effects of Med23 and Runx2 on global gene expression patterns, we performed RNA-seq with total RNA extracted from the calvaria of control and Med23 MSC −/− littermates, as well as WT and Runx2 +/− littermates. Globally, Med23 MSC −/− versus control and Runx2 +/− versus WT revealed a significantly positive correlation in global gene expression ( Fig. 4a ). We next found that downregulated genes in Med23 MSC −/− set presented in a similar pattern in Runx2 +/− set ( Fig. 4b ). In more details, 438 genes were downregulated >1.5-fold in the Med23 MSC −/− set compared with the corresponding control, and 504 genes were downregulated >1.5-fold in the Runx2 +/− set compared with the control and a total of 124 genes overlapped between the 2 groups ( Fig. 4c ). These data further implied that these two molecules may function cooperatively. We then performed a gene ontology (GO) analysis of the set of 1.5-fold significantly downregulated genes from the Med23 MSC −/− sample. The results showed that these genes were enriched for associations with bone development and ossification ( Fig. 4d ). We verified the expression of osteoblast-specific genes in the calvaria from control and Med23 MSC −/− newborns by real-time PCR and found that osteogenic genes such as Osx , Alp , Col1a1 and Ocn were significantly reduced in Med23 MSC −/− mice compared with controls, while Runx2 and Atf4 , another key factor involved in osteogenesis, were unchanged ( Fig. 4e ). Consistently, Von Kossa staining and immunohistochemical analyses of bone tissue sections from E16.5 control and Med23 MSC −/− embryos further confirmed the defects in bone formation and impaired osteoblast differentiation in vivo ( Fig. 4f,g ). Similarly, defects in ossification and decrease in osteogenic gene expression were observed in Med23 ob −/− mice (Supplementary Fig. 3c–e). Both the in vitro and in vivo experiments thus showed that Med23 deletion reduced the expression of multiple Runx2 -target genes while not affecting the expression of Runx2 itself. These observations implied that MED23 may participate in osteoblast differentiation and bone development by controlling RUNX2 activity. 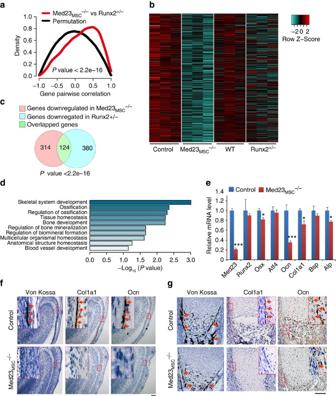Figure 4:Med23regulates expression of genes for osteoblast development. (a) Pair-wise correlation analysis of global gene expression in control versusMed23MSC−/−(Med23MSC−/−set) and in WT versusRunx2+/−(Runx2+/−set). Total RNAs were isolated from calvaria bone of control andMed23MSC−/−newborns and WT andRunx2+/−newborns, followed by RNA sequencing analysis. Kolmogorov–Smirnov (K–S) test was used for testing for correlation betweenMed23MSC−/−set andRunx2+/−set. (b) Heat map analysis of downregulated genes inMed23MSC−/−set andRunx2+/−set. (c) Analysis of downregulated genes (log2fold change>0.5) common toMed23MSC−/− set andRunx2+/−set. (d) Gene ontology (GO) enrichment analysis of downregulated genes (>1.5-fold) inMed23MSC−/−set. (e) Relative expression level of osteogenic marker mRNAs from parietal bones of P2 control andMed23MSC−/−. Data represent means±s.d.t-test, *P<0.05 and ***P<0.001. (f) Sections (4 μm) of skull tissues and (g) sections (4 μm) of tibia bone from E16.5 control andMed23MSC−/−embryos were analysed for bone mineralization by von Kossa staining (left), and for expression ofCol1a1(middle) andOsteocalcin(Ocn) (right) byin situhybridization. Scale bar, 100 μm. Figure 4: Med23 regulates expression of genes for osteoblast development. ( a ) Pair-wise correlation analysis of global gene expression in control versus Med23 MSC −/− ( Med23 MSC −/− set) and in WT versus Runx2 +/− ( Runx2 +/− set). Total RNAs were isolated from calvaria bone of control and Med23 MSC −/− newborns and WT and Runx2 +/− newborns, followed by RNA sequencing analysis. Kolmogorov–Smirnov (K–S) test was used for testing for correlation between Med23 MSC −/− set and Runx2 +/− set. ( b ) Heat map analysis of downregulated genes in Med23 MSC −/− set and Runx2 +/− set. ( c ) Analysis of downregulated genes (log 2 fold change>0.5) common to Med2 3 MSC −/− set and Runx2 +/− set. ( d ) Gene ontology (GO) enrichment analysis of downregulated genes (>1.5-fold) in Med23 MSC −/− set. ( e ) Relative expression level of osteogenic marker mRNAs from parietal bones of P2 control and Med23 MSC −/− . Data represent means±s.d. t -test, * P <0.05 and *** P <0.001. ( f ) Sections (4 μm) of skull tissues and ( g ) sections (4 μm) of tibia bone from E16.5 control and Med23 MSC −/− embryos were analysed for bone mineralization by von Kossa staining (left), and for expression of Col1a1 (middle) and Osteocalcin ( Ocn ) (right) by in situ hybridization. Scale bar, 100 μm. Full size image Med23 modulates Runx2 activity as a cofactor We next set out to investigate whether MED23 controls the transcriptional activity of Runx2 . To this end, we infected murine C3H10T1/2 embryonic fibroblasts with retroviruses expressing control or Med23 knockdown shRNAs and then transfected the stable cells with a luciferase reporter driven by the Ocn promoter (OC1050-Luc), which is a prototypical Runx2-target gene promoter that is widely used as a tool to study the molecular regulation of osteoblast development [24] . In the absence of MED23, RUNX2-dependent activation of the Ocn promoter was significantly inhibited ( Fig. 5a ). The Ocn promoter harbours two binding sites: OSE2 and OSE1, which are specifically bound by Runx2 and ATF4, respectively [25] . To discriminate the effects of Med23 deficiency on the two key factors, we performed the luciferase reporter assay with either 6XOSE2-Luc or 6XOSE1-Luc in control and Med23 shRNA knockdown cells. Med23 deficiency specifically impaired the Runx2-driven activation of 6XOSE2-Luc but did not affect the ATF4-driven activation of 6XOSE1-Luc, suggesting a specific connection between Med23 and Runx2 ( Fig. 5b,c ). To further verify the specific regulation of RUNX2 activity by MED23, we performed a titration experiment with low and high doses of MED23 co-transfected with the OC1050-Luc reporter, which showed that RUNX2 activity was repressed gradually with increasing dose of MED23 ( Fig. 5d ). The repressive effect on RUNX2 activity by overexpression of MED23 was also confirmed by 6XOSE2-Luc reporter system (Supplementary Fig. 7a). By contrast, overexpression of MED23 did not affect ATF4 activity ( Fig. 5d and Supplementary Fig. 7b). RUNX2 activity was quenched by high level overexpression of MED23 probably in that the exogenous MED23 may compete with endogenous MED23 within the Mediator complex to prevent the transcription factor Runx2 from recruiting the Mediator complex. 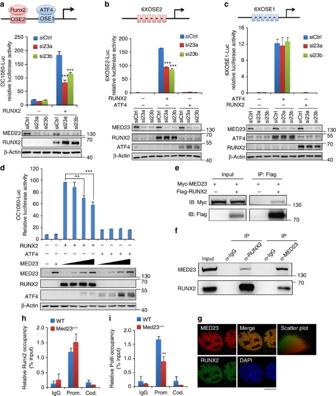Figure 5: Regulation of RUNX2 transcriptional activity by MED23. (a–c) Effect ofMed23deficiency on Runx2-mediated activation of theosteocalcintested with luciferase expression report systems (a) OC1050-Luc, (b) 6XOSE2-Luc and (c) 6XOSE1-Luc. Luciferase assay was performed in control andMed23knockdown C310T1/2 cells.n=3 for each group, all data represent means±s.d.t-test, ***P<0.001 (d) Effects of an increasing amount of MED23 on transcriptional activity of Runx2 in C310T1/2 cells with the OC1050-Luc report system. Below is the western blot analysis of MED23 levels in the lysates.n=3 for each group, all data represent means±s.d.t-test. **P<0.01, ***P<0.001 (e) Co-immunoprecipitation (Co-IP) of MED23 with Flag-RUNX2. Flag-RUNX2 expressing plasmid was co-transfected with Myc-Med23 into 293T cells. Whole cell lysate was used for immunoprecipitation and then immunoblotting with indicated antibodies. (f) Physical interaction between endogenous RUNX2 and MED23. Co-IP experiment was performed in BMP2-stimulated MC3T3E1 cells. Whole cell lysate was used for immunoprecipitation with anti-RUNX2 or anti-MED23, followed by detection with indicated antibodies by western blot. (g) Co-localization assay in primary osteoblast cells. Cells were IF stained with antibodies against MED23 and RUNX2 after stimulated with BMP2 for 24 h. Scale bar, 10 μm. The scatter plot showed FITC and RRX emission intensities were plotted onx- andy-axes, respectively. Co-localization was analysed by the Volocity software, which showed the coefficient for co-localization of 0.786±0.003 (Pearson’s correlation coefficient). (h,i) ChIP assay for occupation of RUNX2 (h) or Pol II (i) on the promoter of Osteocalcin. Immortalized WT andMed23−/−bone marrow-derived mesenchymal cells were cultured in osteogenic medium for 6 days, followed by fixation and lysation. Chromatin from cell lysates was immunoprecipited with anti-RUNX2 or anti-Pol II and quantified by RT–PCR. ‘Prom’ represents the promoter region and ‘Cod’ represents the coding region.n=3 for each group, all data represent means±s.d.t-test, **P<0.01. Figure 5: Regulation of RUNX2 transcriptional activity by MED23. ( a – c ) Effect of Med23 deficiency on Runx2-mediated activation of the osteocalcin tested with luciferase expression report systems ( a ) OC1050-Luc, ( b ) 6XOSE2-Luc and ( c ) 6XOSE1-Luc. Luciferase assay was performed in control and Med23 knockdown C310T1/2 cells. n =3 for each group, all data represent means±s.d. t -test, *** P <0.001 ( d ) Effects of an increasing amount of MED23 on transcriptional activity of Runx2 in C310T1/2 cells with the OC1050-Luc report system. Below is the western blot analysis of MED23 levels in the lysates. n =3 for each group, all data represent means±s.d. t -test. ** P <0.01, *** P <0.001 ( e ) Co-immunoprecipitation (Co-IP) of MED23 with Flag-RUNX2. Flag-RUNX2 expressing plasmid was co-transfected with Myc-Med23 into 293T cells. Whole cell lysate was used for immunoprecipitation and then immunoblotting with indicated antibodies. ( f ) Physical interaction between endogenous RUNX2 and MED23. Co-IP experiment was performed in BMP2-stimulated MC3T3E1 cells. Whole cell lysate was used for immunoprecipitation with anti-RUNX2 or anti-MED23, followed by detection with indicated antibodies by western blot. ( g ) Co-localization assay in primary osteoblast cells. Cells were IF stained with antibodies against MED23 and RUNX2 after stimulated with BMP2 for 24 h. Scale bar, 10 μm. The scatter plot showed FITC and RRX emission intensities were plotted on x - and y -axes, respectively. Co-localization was analysed by the Volocity software, which showed the coefficient for co-localization of 0.786±0.003 (Pearson’s correlation coefficient). ( h , i ) ChIP assay for occupation of RUNX2 ( h ) or Pol II ( i ) on the promoter of Osteocalcin. Immortalized WT and Med23 −/− bone marrow-derived mesenchymal cells were cultured in osteogenic medium for 6 days, followed by fixation and lysation. Chromatin from cell lysates was immunoprecipited with anti-RUNX2 or anti-Pol II and quantified by RT–PCR. ‘Prom’ represents the promoter region and ‘Cod’ represents the coding region. n =3 for each group, all data represent means±s.d. t -test, ** P <0.01. Full size image Cooperative activation of the Ocn promoter by MED23 and RUNX2 led us to examine the physical interaction between the two molecules. We transfected 293T cells with tagged Runx2 and Med23 and performed a co-immunoprecipitation (co-IP) assay, which revealed that MED23 physically associated with RUNX2 ( Fig. 5e ). Consistent with these results, endogenous RUNX2 and MED23 interacted in differentiated MC3T3E1 osteoblastic cells ( Fig. 5f ). The interaction with MED23 was mediated via the Runt and PST domains of RUNX2 (Supplementary Fig. 8a,b). GST pull-down assay implied that MED23/RUNX2 interaction was likely direct (Supplementary Fig. 8c). Moreover, immunofluorescence staining showed that these two proteins largely colocalized in the nucleus ( Fig. 5g ). As gene transcription involves a key step in which the activators work with the Mediator complex to recruit RNA Pol II to the gene promoters, we next used a chromatin IP (ChIP) assay to test whether Med23 deletion affected the recruitment of RNA Pol II by RUNX2 and the binding of RUNX2 to its target’s promoter. The result showed that the occupancy of Pol II at the promoter of Ocn , a direct target gene of Runx2 , was markedly decreased in the absence of MED23 while RUNX2 occupancy did not alter, suggesting that Med23 deficiency impaired the recruitment of Pol II to the promoter of Runx2-target osteogenic marker genes ( Fig. 5h ). Taken together, these results suggest that the Mediator subunit MED23 acts as a coactivator of Runx2 to regulate osteoblast differentiation. Med23 genetically interacts with Runx2 during osteogenesis Based on the in vitro findings described above, we next questioned whether MED23 synergized with RUNX2 in vivo . We hypothesized that if MED23 acts together with RUNX2 to regulate osteoblast activity, then deletion of Med23 in parallel with Runx2 haploinsufficiency in vivo should aggravate the skeletal defects observed in Runx2 +/− mice. To test this hypothesis and since disruption in single copy of Med23 did not reduce the protein level of MED23, we crossed Med23 MSC −/− mice with Med23 fl/fl /Runx2 +/− mice and analysed the skeletal phenotypes of E16.5 embryos by alcian blue/ARS double staining. As shown in Fig. 6a , both Med23 fl/fl /Runx2 +/− mice and Med23 MSC −/− mice showed the previously reported CCD-like skeletal abnormalities observed in heterozygous Runx2 mutant mice [8] , [10] . Runx2 +/− / Med23 MSC −/− mice displayed significant bone defects, including delayed ossification of the fontanelles and hypoplasia of the clavicles ( Fig. 6a ). Furthermore, Von Kossa staining revealed reduced ossification of the long bones of E16.5 Runx2 +/− and Med23 MSC −/− mice compared with control mice. However, Runx2 +/− / Med23 MSC −/− compound mutant mice displayed a more severe reduction in ossification ( Fig. 6b ). Consistent with the reduced Von Kossa staining, the expression of Ocn was decreased significantly in the Runx2 +/− / Med23 MSC −/− compound mutant mice compared with the Runx2 +/− mice and Med23 MSC −/− mice ( Fig. 6c ). Taken together, these data indicate a genetic interaction between Med23 and Runx2 and provide in vivo verification that MED23 can regulate osteoblast function via cooperation with RUNX2. 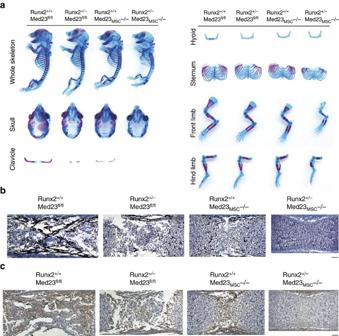Figure 6: Med23 genetically associates with Runx2. (a) Skeletons of E16.5 mice (Runx2+/+Med23fl/fl,Runx2+/−Med23fl/fl,Runx2+/+Med23MSC−/−,Runx2+/−Med23MSC−/−) were double stained by alizarin red/alcian blue. (b) Von Kossa staining of humeri from E15.5 mice (Runx2+/+Med23fl/fl,Runx2+/−Med23fl/fl,Runx2+/+Med23MSC−/−,Runx2+/−Med23MSC−/−). Scale bar, 100 μm. (c) Immunohistochemistry assay for expression ofOsteocalcin(Ocn) in E16.5 mice (Runx2+/+Med23fl/fl,Runx2+/−Med23fl/fl,Runx2+/+Med23MSC−/−,Runx2+/−Med23MSC−/−). Scale bar, 100 μm. Figure 6: Med23 genetically associates with Runx2. ( a ) Skeletons of E16.5 mice ( Runx2 +/+ Med23 fl/fl , Runx2 +/− Med23 fl/fl , Runx2 +/+ Med23 MSC −/− , Runx2 +/− Med23 MSC −/− ) were double stained by alizarin red/alcian blue. ( b ) Von Kossa staining of humeri from E15.5 mice ( Runx2 +/+ Med23 fl/fl , Runx2 +/− Med23 fl/fl , Runx2 +/+ Med23 MSC −/− , Runx2 +/− Med23 MSC −/− ). Scale bar, 100 μm. ( c ) Immunohistochemistry assay for expression of Osteocalcin ( Ocn ) in E16.5 mice ( Runx2 +/+ Med23 fl/fl , Runx2 +/− Med23 fl/fl , Runx2 +/+ Med23 MSC −/− , Runx2 +/− Med23 MSC −/− ). Scale bar, 100 μm. Full size image The present study provides several lines of evidence that Med23 is required for osteoblast differentiation and bone development. Homozygous loss of Med23 in mesenchymal progenitors resulted in prominent defects in bone development, including hypoplasia of the clavicles, retarded ossification of the cranial bones and reductions in the trabecular bone and overall bone mass. Furthermore, Med23 conditional knockout in preosteoblasts largely recapitulated the characteristics of Med23 MSC −/− mice. Phenotypic analysis showed that Med23 deficiency affected both intramembranous and endochondral bone formation. In vitro differentiation experiments indicated that the defective osteogenesis happened in a cell-autonomous manner. In contrast to the impaired osteoblast development, the presence of multinucleated osteoclasts in the mineralized cartilage matrix of Med23 -deficient mice indicated that osteoclast differentiation occurred normally. MSCs can differentiate into different lineages, including osteoblasts, adipocytes, chondrocytes and myocytes [1] , [2] . Different transcription factors have been shown to specify distinct cell fates. In addition to the function of Runx2 in osteoblast differentiation, PPARγ , Sox9 and MyoD drive MSCs to differentiate into adipocytes, chondrocytes and myocytes, respectively [7] , [8] , [26] , [27] , [28] . The role of the Mediator complex in PPARγ -mediated adipogenesis has been established by observing a direct interaction between MED1 and PPARγ [13] . For Sox9 , studies from the zebra fish model indicated that Trap230/MED12 can function as a coactivator for SOX9 during cartilage development, with Trap230 / Med12 mutant zebra fish strikingly resembling the Sox9 mutant phenotype [29] . Our previous study demonstrated that MED23 represses smooth muscle cell differentiation while facilitating adipocyte differentiation in multipotent MSCs [16] , indicating that a single Mediator complex subunit is able to regulate the differentiation of MSCs into various cell lineages, either positively or negatively, by cooperating with lineage-specifying transcription factors such as ELK1 and MAL. To date, there have been no reports of a direct role for the Mediator complex in RUNX2 function. Our study demonstrated that MED23 can act together with RUNX2 to drive osteoblast differentiation. To the best of our knowledge, this is the first report of a direct role for the Mediator complex in modulating RUNX2 function. We provide evidence that the Mediator complex subunit MED23 partially regulates the transcriptional activity of RUNX2 and is required for osteoblast differentiation and bone development. First, homozygous loss of Med23 in mesenchymal progenitors resembled the bone phenotype of Runx2 heterozygous mice, resulting in prominent defects in bone development, with hypoplasia of the clavicles, retarded ossification of the cranial bones and reduction in the trabecular bone and overall bone mass. Moreover, Med23 conditional knockout in preosteoblasts largely recapitulated the characteristics of Med23 MSC −/− mice, with abnormalities in multiple skeletal elements. Interestingly, Med23 deficiency did not alter RUNX2 expression but instead caused the downregulation of multiple Runx2 -regulated genes, such as Osx and Ocn . Reporter assays revealed that Med23 deficiency impaired Runx2 transcriptional activity but did not affect the activity of ATF4, another key regulator of osteoblast differentiation. Biochemical analyses further established the physical association between RUNX2 and MED23. Finally, Med23 deletion further aggravated the defective skeletal phenotype of Runx2 +/− mice. In addition to the function in osteoblasts, Runx2 is also found to control the maturation of chondrocytes through Runx2 conditional knockout in chondrocytes by Col2a1-Cre [30] , [31] . Histological analysis of tibia showed that chondrocytes were arrested during terminal maturation in Med23 MSC −/− mice compared with control littermates as evidenced by less endochondral ossification and smaller hypertrophic chondrocytes in Med23 MSC −/− mice (Supplementary Fig. 10a–c). All the results described above provide in vivo genetic evidence that MED23 is a cofactor of RUNX2. Runx2 mutations are known to underlie human CCD, an autosomal-dominant heritable skeletal disease that is typically characterized by open or delayed closure of calvarial fontanelles and clavicle hypoplasia [9] , [32] , [33] . This phenotype can be reproduced in heterozygous Runx2 mutant mice [10] . More precisely, a 70% reduction in Runx2 levels also generates the CCD phenotype in mice [34] . Indeed, human bone marrow-derived MSCs with Med23 deficiency were retarded to differentiate into osteoblasts, which might imply that MED23 plays a role in human skeletal development and its mutation may relate to human bone diseases (Supplementary Fig. 9). In addition, the dysregulation of Runx2 activity through manipulation of numerous nuclear factors, for example, TAZ, MAF and Satb2, causes abnormal osteoblast differentiation and bone development [11] , [35] , [36] . These studies indicate that the Runx2 -dependent transcriptional output is under fine surveillance via the cooperation of many factors. Our study demonstrated that the Mediator subunit MED23 acts as a cofactor of RUNX2 in the regulation of osteoblast differentiation and bone development, providing an insight into the regulation of RUNX2 activity and skeletal dysplasias such as CCD. Mice Med23 -floxed mice were generated by homologous recombination [16] , [17] . Briefly, the exons 5–7 were flanked by two loxP sites. After targeting vector delivery, ES cells were screened by PCR. Med23 -floxed mice were backcrossed with C57/BL6J mice for at least six generations. Prx1-Cre and Osx-Cre-ER mice were purchased from the Jackson Laboratory. Runx2 +/− mice were kindly provided by Professor Laurie Glimcher’s lab. All mice were maintained under specific pathogen-free conditions. All animal experimental procedures were approved by the Institutional Animal Care and Research Advisory Committee of the Shanghai Institute of Biochemistry and Cell Biology. Analysis of bone phenotypes Skeletal preparations were double stained with alcian blue and ARS [8] , [10] . Briefly, embryos or newborns were eviscerated and the skin was removed. After fixation with 95% ethanol for 3 days, embryos or newborns were stained for 3 days in Alcian blue solution. Then they were fixed and cleared with 95% ethanol for three times and each 1.5 h, followed by treatment of 2% KOH for 3–4 h. After stained with ARS solution for 3–4 h, skeletons were cleared in 1%KOH/20% glycerol. For histological analysis, bone tissues were fixed in 4% paraformaldehyde (PFA) and then embedded in paraffin. For embryonic mice, 4 μm tissue sections were used for Von Kossa staining, DIG labelled in situ hybridization (Roche) and immunohistochemical staining (Dako). For postnatal mice, bone tissues were fixed in 4% PFA and decalcified for 2 weeks prior to paraffin embedding. Tissue sections (4 μm) were used for TRAP staining according to the standard protocol. Measurement of PINP concentrations We determined serum concentrations of PINP using the mouse PINP EIA kit (Immunodiagnostic Systems) according to the instructions provided. Micro CT analysis Mouse hind limbs were harvested, soft tissues were removed and the remaining tissues were stored in 70% ethanol. Scanning was performed with a Skyscan1076 instrument, and 36 slides (18 μm each) immediately below the growth plate in the distal metaphysis of the femur were used for quantification of the bone parameters. Cell culture C310T1/2 (ATCC) and 293T (ATCC) cells were maintained in DMEM containing 10% FBS. MC3T3E1 (ATCC) cells were maintained in Minimum Essential Medium α (α-MEM) containing 10% FBS. MSCs were isolated from bone marrow samples of 6- to 8-week-old mice and cultured in α-MEM containing 15% FBS. All cells were cultured in a 5% CO 2 humidified incubator at 37 °C. For the c.f.u.-F assay, 2 × 10 6 bone marrow-derived MSCs or 1 × 10 2 osteoblast cells from calvaria were plated on each well of a six-well plate, cultured for 2 weeks and then fixed in 4% PFA and stained with 0.5% crystal violet, followed by counting the stained colonies. For in vitro osteoblast differentiation, MSCs were cultured in osteogenic medium (10% FBS with 50 μg ml −1 ascorbic acid, 10 nM dexamethasone and 10 mM β-glycerophosphate) and subjected to ALP staining on day 7 and ARS staining on day 21. Human bone marrow-derived MSCs were cultured and induced to differentiate into osteoblasts according to the protocol from ScienCell. Transient transfection and luciferase reporter assay C3H10T1/2 cells were seeded overnight at 4 × 10 4 cells per well into a 24-well plate and transfected by Lipofectamine 2000 (Life Technologies) with a luciferase reporter plasmid and pRL-TK (Promega) along with various expression constructs, as indicated. All wells were supplemented with control empty expression vector plasmids to keep the total amount of DNA constant. At 36–48 h post transfection, the cells were harvested and subjected to dual-luciferase reporter assays according to the manufacturer’s protocol (Promega). IP and immunoblotting 293T cells were seeded at 6 × 10 6 cells per 10 cm dish and cultured overnight. At 36–48 h after transfection with Lipofectamine 2000, cells were harvested and lysed in lysis buffer (1% NP-40, 10% glycerol, 135 mM NaCl, 20 mM Tris, pH 8.0) supplemented with protease inhibitors. Lysates were subjected to IP with anti-Flag antibodies (M2, Sigma) at 4 °C overnight, followed by washing in lysis buffer, SDS–PAGE electrophoresis and immunoblotting with the indicated antibody (1:2,000, anti-Myc , Sigma). To investigate endogenous protein–protein interactions, MC3T3E1 cells were cultured for 4 days in α-MEM with 10% FBS supplemented with 100 ng ml −1 BMP2, 50 μg ml −1 ascorbic acid and 10 mM β-glycerophosphate. Two hours prior to harvest, MG132 (10 μM, Sigma) was added to all cultures. Harvested cells were subjected to lysis and IP with anti-RUNX2 (Sigma), anti-MED23 (Novus) or control IgG, followed by washing in lysis buffer, SDS–PAGE electrophoresis and immunoblotting with the indicated antibody (Anti-MED23, 1:1,000, BD Biosciences; anti-Runx2, 1:1,000, MBL). Primary bone marrow MSCs or bone tissues were lysed in RIPA buffer (50 mM Tris pH7.4, 150 mM NaCl, 1% Triton X-100, 1% sodium deoxycholate, 0.1% SDS) in presence of protease inhibitors. Whole cell lysate were centrifuged and then subjected to western blots according to standard protocols. Uncropped results for all western blots are shown in Supplementary Fig. 11. In vitro interaction assay GST or GST-RUNX2 recombined proteins were expressed in Escherichia coli BL21, followed by purification according to the instructions of the manufacturer (GE). His-Flag-MED23 was expressed using the Bac-to-Bac baculovirus expression system and purified by Ni-NTA agarose beads (Invitrogen). Purified GST or GST-Runx2 was incubated with purified MED23 and subjected to GST pull-down experiment . The bound proteins were analysed by SDS–10% PAGE and immunoblotting with indicated antibodies (Anti-GST, 1:1,000, Santa Cruz; anti-MED23, 1:1,000). Immunofluorescence staining and co-localization analysis Primary osteoblast cells were plated on cover slips for 24 h in α-MEM with 10% FBS with BMP2 (100 ng ml −1 ) prior to staining. After removal of culture media, cells were washed with PBS, fixed in 4% PFA, permeabilized with 0.2% Triton X-100 for 10 min and then blocked with 2% BSA in PBS for 1 h. Anti-MED23 (1:100) and anti-RUNX2 (1:200) primary antibodies were diluted in the blocking solution and applied overnight at 4°C. After PBS wash for three times, secondary antibodies (Jackson Laboratory) were diluted (1:100) in blocking buffer and applied for 1 h at room temperature. After PBS wash for three times, nuclei were stained with DAPI (1:4,000) for 4 min. Co-localization analysis were performed using Volocity Software (PerkinElmer). Real-time PCR analysis Total RNA was isolated from bone tissue or cells with TRIzol reagent (Life Technologies). Complementary DNA was generated using M-MLV reverse transcription kit (Promega). Real-time PCR was conducted in triplicate with SYBR Premix Ex Taq (Takara). The level of the endogenous mRNA was normalized to the level of Gapdh mRNA using the 2 −ΔCT method. Specific primer sequences are listed in the Supplementary Table 1. ChIP assay Cells were cross-linked with 1% formaldehyde in culture media for 10 min at room temperature, followed by adding 0.125 M glycine to quench the cross-linking. Cells were washed and scraped in cold PBS and harvested in ChIP lysis buffer (50 mM Tris-HCl, pH 7.4, 1% SDS, 10 mM EDTA). Cell lysates were then sonicated to shear chromatin. After that, cell lysates were centrifuged and 100 μl supernatant was diluted with 900 μl dilution buffer (16.7 mM Tris-HCl, pH 8.0, 0.01% SDS, 1.1% Triton X-100, 1.2 mM EDTA, 167 mM NaCl) and then incubated with 2 μg anti-RUNX2 or 2 μg anti-Pol II (Santa Cruz) or non-immune Rabbit IgG overnight at 4° C. About 20 μl Protein G magnetic beads (Life technologies) were added for another 4 h on a rotating wheel. Chromatin then was immunoprecipitated, decrosslinked at 65 °C and treated with Proteinase K. Precipitated DNA was extracted and quantified by real-time PCR. All values were normalized to input. Specific primer sequences were listed in Supplementary Table 1. Retrovirus infection Retroviruses expressing RNA interference (RNAi) oligonucleotides were generated by transfection of recombinant pSiren-RetroQ and pCL10A1 helper plasmids into 293T cells using Lipofectamine 2000. Culture media were changed 24 h after transfection and the supernatants containing retroviruses were harvested 48 h later and passed through a 0.45-μm filter. Filtered supernatants were supplemented with 6 μg ml −1 polybrene and added to the cells grown in six-well plates for centrifugation at 2,500 r.p.m. for 1.5 h at 30 °C. About 24 h after spin infection, infected cells were then selected in the presence of puromycin: primary MSCs at 5 μg ml −1 and C3H10T1/2 at 8 μg ml −1 . The RNAi oligo sequences are listed in Supplementary Table 2. RNA-Seq and GO analysis Total RNA was isolated with TRIzol from the parietal bone of P2 control mice ( n =3) and Med23 MSC −/− littermates ( n =3) and from the parietal bone of P2 WT mice ( n =3) and Runx2 +/− mice ( n =3). Complementary DNA library preparation and sequencing were performed according to the Illumina standard protocol. GO analysis was performed with the DAVID online tool. Top GO categories were selected according to the P values. RNA-seq data in this study have been deposited at Gene Expression Omnibus (GEO) ( http://www.ncbi.nlm.nih.gov/gen/ ) under accession ID GSE 77007. Statistical analysis Statistical analyses were performed with two-tailed, unpaired Student’s t -test. Kolmogorov–Smirnov test was used to test for comparing cumulative distributions of two data sets ( Fig. 4a ). Accession codes: RNA-seq data has been deposited in the Gene Expression Omnibus (GEO) Data Bank ( http://www.ncbi.nlm.nih.gov/gen/ ) under accession code ID GSE77007 . How to cite this article: Liu, Z. et al . Mediator MED23 cooperates with RUNX2 to drive osteoblast differentiation and bone development. Nat. Commun. 7:11149 doi: 10.1038/ncomms11149 (2016).